Arrayed lipid bilayer chambers allow single-molecule analysis of membrane transporter activity Nano- to micron-size reaction chamber arrays (femtolitre chamber arrays) have facilitated the development of sensitive and quantitative biological assays, such as single-molecule enzymatic assays, digital PCR and digital ELISA. However, the versatility of femtolitre chamber arrays is limited to reactions that occur in aqueous solutions. Here we report an arrayed lipid bilayer chamber system (ALBiC) that contains sub-million femtolitre chambers, each sealed with a stable 4-μm-diameter lipid bilayer membrane. When reconstituted with a limiting amount of the membrane transporter proteins α-hemolysin or F 0 F 1 -ATP synthase, the chambers within the ALBiC exhibit stochastic and quantized transporting activities. This demonstrates that the single-molecule analysis of passive and active membrane transport is achievable with the ALBiC system. This new platform broadens the versatility of femtolitre chamber arrays and paves the way for novel applications aimed at furthering our mechanistic understanding of membrane proteins’ function. The membrane proteins responsible for the transport of substrate molecules across biomembranes play pivotal physiologic roles such as nutrient uptake, secretion of proteins or signal molecules, exclusion of waste or exogenous compounds and energy transduction [1] . Due to their physiological importance, transporters are important pharmacological targets [2] , [3] . Although extensive studies have been conducted to elucidate the mechanisms of transport, quantitatively and reproducibly measuring the activity of transporters in a high-throughput format has remained difficult due to the complexity of membrane system formation processes. Transporter activity is usually measured by reconstituting transporter molecules into liposomes that contain indicator dyes as substrates. Although this approach is versatile and relatively easy, quantitative analysis is generally not possible due to the heterogeneity in liposome shape and the unknown number of active transporters ultimately reconstituted into each liposome. Electrochemical measurements using transporters reconstituted into a planar bilayer formed on the orifice of a solid or polymer sheet and separating two buffer chambers is another option. When a substrate molecule is charged, the transport activity is detected as an electric current. However, the transport rate of active transporters is generally far below that of ion channels or pore-forming transporters, which passively translocate ions or small molecules down the electrochemical gradient at rates in excess of 10 7 s −1 . Therefore, electrochemical analysis suffers the requirement for the reconstitution of several transporter molecules. A method for the quantitative measurement of active transporters and transporter activity at the single-molecule level is thus highly anticipated. In an attempt to analyse transporter activity at the single-molecule level using optical methods, microsystems for micron-sized reactors sealed with lipid bilayers (lipid bilayer chambers) have been developed where transport is measured based on substrate accumulation in the chamber [4] , [5] , [6] . Although these methods have improved detection, single-molecule analysis of active transporters has not yet been achieved due to the technical difficulties of forming bilayer chambers with high reproducibility in a high-throughput manner. Here we address this issue by developing a microsystem that forms arrayed lipid bilayer chambers (ALBiCs) to achieve highly sensitive, quantitative analysis of active transporter proteins. Formation of lipid bilayer membranes on microchambers We fabricated a device that had more than 100,000 through-hole structures on a carbon–fluorine hydrophobic polymer (CYTOP, Asahi-glass, Japan) on a hydrophilic glass substrate (32 mm × 24 mm), as previously reported ( Fig. 1b ) [7] . To enhance sensitivity, the through-hole structures (7 fL, φ =4 μm and h =500 nm) were utilized as microchambers of much smaller size than previously reported ( Fig. 1 ) [4] , [8] , [9] . For exchange of the sample solution, a flow cell was constructed from the microchamber array patterned on a cover slip, spacer sheet and CYTOP-coated glass block, which had an access port for sample injection ( Fig. 1a ). Lipid membranes were formed on the top orifice of the microchambers via sequential injection of liquid from the access port ( Fig. 2a ). First, an aqueous solution containing fluorescent reporter dyes was infused into the flow cell. Then, a lipid solution containing 4 mg ml −1 lipid (a 1:1 [w:w] mixture of 1,2-dioleoyl- sn -glycero-3-phosphoethanolamine (DOPE) and 1,2-dioleoyl- sn -glycero-3-phosphoglycerol (DOPG)) in chloroform was infused to flush away the first aqueous solution. After flushing, water-in-organic solvent droplets were formed in the individual chambers. Then, a second aqueous solution was infused to flush the lipid solution. The residual lipids formed a lipid membrane on the opened orifice of the microchambers ( Fig. 2b ), with an efficiency of >99% (number of sealed chambers: 112,996 versus total number of chambers: 113,736, yielding 99.3% efficiency). Notably, various types of organic solvents and lipid molecules could be used for membrane formation, for example, decane, hexadecane, soy-bean lipid and total Escherichia coli lipid ( Supplementary Fig. 1 ), demonstrating the versatility of the ALBiC system. Bright-field observation showed circular interference patterns in the individual chambers after the lipid membrane formation ( Supplementary Fig. 2B ), while a clear circular pattern was not observed before membrane formation ( Supplementary Fig. 2A ). This interference pattern is a characteristic optical feature of thin lipid bilayer formation, termed the Plateau–Gibbs border [10] , [11] . Thus, bright-field observation supported the formation of lipid bilayers in the ALBiC system. Lipid bilayer formation was further confirmed from the activity of membrane transporters (see below), which were not functional unless the lipid membrane became as thin as the membrane-spanning structure of these transporter proteins (4–5 nm). 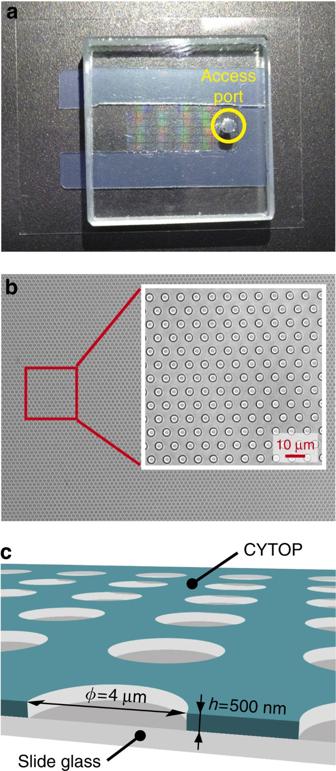Figure 1: Microchamber arrays for lipid bilayer membrane formation. (a) Fabricated microdevices, where the substrate (~100,000 arrays of hydrophilic-in-hydrophobic structures) was assembled with CYTOP-coated cover glass having an access port for sample injection. (b) The bright-field image of through-hole structures of the carbon–fluorine hydrophobic polymer on a hydrophilic glass substrate. (c) Illustration of a fabricated structure (diameter, 4 μm; thickness, 500 nm). Figure 1: Microchamber arrays for lipid bilayer membrane formation. ( a ) Fabricated microdevices, where the substrate (~100,000 arrays of hydrophilic-in-hydrophobic structures) was assembled with CYTOP-coated cover glass having an access port for sample injection. ( b ) The bright-field image of through-hole structures of the carbon–fluorine hydrophobic polymer on a hydrophilic glass substrate. ( c ) Illustration of a fabricated structure (diameter, 4 μm; thickness, 500 nm). 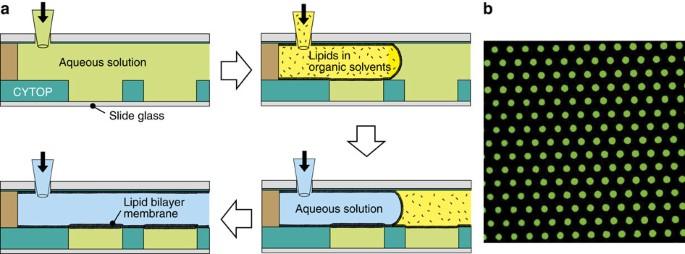Figure 2: Formation of a lipid bilayer membrane. (a) Schematic illustration of lipid membrane formation processes. In these processes, unilamellar lipid bilayer membranes formed on the inlet of individual chambers. (b) Fluorescent image of Alexa 488 encapsulated into microchambers sealed by lipid membranes. Full size image Figure 2: Formation of a lipid bilayer membrane. ( a ) Schematic illustration of lipid membrane formation processes. In these processes, unilamellar lipid bilayer membranes formed on the inlet of individual chambers. ( b ) Fluorescent image of Alexa 488 encapsulated into microchambers sealed by lipid membranes. Full size image The ALBiCs formed in this study were hermetically sealed for stable retention of the solute, as confirmed by fluorescence recovery after photobleaching. ALBiCs were filled with the fluorescent dye Alexa 488 ( Supplementary Fig. 3 ) or RhP-M ( Supplementary Figs 4–6 ) [12] , which was used as a pH-sensitive dye for analysis of the transport activity of F 0 F 1 -ATP synthase. Fluorescent images were recorded with 100-s intervals using a confocal microscope ( Supplementary Figs 7A and 8A ). Notably, some RhP-M molecules bound nonspecifically to the chamber wall due to its hydrophobicity, exhibiting ring-like shapes in fluorescent images ( Supplementary Fig. 4 ). Therefore, we selectively analysed the fluorescent profile of RhP-M at the centre of the chamber, omitting the fluorescent signal localized along the chamber wall. Using the laser-scanning system of the confocal microscope, one of the chambers was selectively photobleached ( Supplementary Figs 7A and 8A ). A subsequent recording of the fluorescence intensity showed that the bleached chamber did not recover its original fluorescence, suggesting that the dye did not diffuse within the 2-h observation period ( Supplementary Figs 7B and 8B ). Thus, the crosstalk between the chambers was negligible, supporting the integrity of the hermetic seal generated by the lipid membrane. A similar experiment using different lipid compositions, that is, soy lipid and E. coli lipid, confirmed the robustness of hermetic seal by the lipid membrane in ALBiC ( Supplementary Fig. 7C,D ). We also tested the possibility of ion leakage from the chambers ( Supplementary Figs 9 and 10 ). For proton leakage tests, acidic buffer (pH 5) was encapsulated in the chambers with the fluorescent pH indicator RhP-M ( Supplementary Fig. 9 ), which exhibits increased fluorescence intensity on acidification ( Supplementary Figs 5 and 6 ). The buffer in the flow cells was then exchanged with neutral buffer (pH 7.1) under a microscope ( Supplementary Fig. 9 ). Before and after the buffer exchange, the fluorescence intensity of RhP-M was stable, demonstrating that the hermetic seal of the ALBiC prevented ion leakage for 2 h. A similar experiment confirmed that Ca 2+ also did not leak from the sealed chamber ( Supplementary Fig. 10 ). Single-molecule analysis of passive membrane transport We conducted passive transport assays using α-hemolysin ( Fig. 3a ), a toxic membrane protein that binds to lipid bilayer membranes and forms transmembrane nanopores [13] ( φ =1–2 nm) that have been used as various biomedical sensors, for example, nanopore-based DNA sequencing [14] . While monomers of α-hemolysin are soluble in water, once bound onto a lipid bilayer, α-hemolysin assembles into a heptameric ring and forms a nanopore at the centre. Because α-hemolysin acts as a passive transporter only when the nanopore penetrates the lipid membrane, the transport activity of α-hemolysin is often used to confirm the formation of a thin lipid bilayer (4–5 nm). To confirm the formation of a thin lipid bilayer in the ALBiC system, α-hemolysin solution was introduced into the flow channel of ALBiCs. A fluorescent dye (Alexa 488) was encapsulated in the chambers as the transport substrate before the α-hemolysin injection. 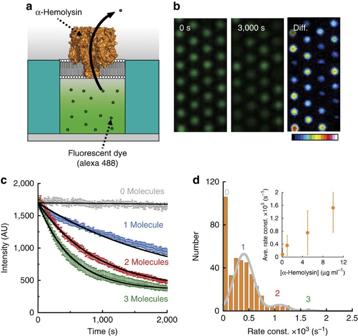Figure 3: Passive transport of fluorescent dye by α-hemolysin. (a) Schematic illustration of passive transport of α-hemolysin reconstituted into ALBiCs. The fluorescent dye (Alexa 488) diffused out from the chamber via the hole on the membrane formed by α-hemolysin. (b) Fluorescent images of the passive transport activity in the chambers. The images were recorded just after α-hemolysin injection (left panel) and 3,000 s later (middle panel). The right panel, diff., shows the intensity difference between these two images in the form of a colour gradient. (c) Continuous recording of the passive transport activity of 1 μg ml−1α-hemolysin. The average of four representative chambers containing 0 α-hemolysin pores, that of four chambers containing 1 α-hemolysin pore, that of four chambers containing 2 α-hemolysin pores and that of four chambers containing 3 α-hemolysin pores were plotted as grey, blue, red and green, respectively. Over the study period, activity was observed as a continuous decrease in the fluorescence concentration, indicating that α-hemolysin was not inactivated temporarily. Solid lines represent the fittings with the single exponential decay:y=C1exp(−k ˙ t)+C2, wherekis the rate constant of passive transport. Error bars represent s.d. (d) In the histogram, the number of chambers is plotted versus the rate constant of passive transport,k. The four peaks can be attributed to occupancies of 0, 1, 2 or 3 α-hemolysin pores per chamber. They were fitted to a sum of Gaussians. The inset is the average (Ave.) rate constant (const.) against the concentration of α-hemolysin in the flow cell. The grey solid line represents the linear fitting with a correlation coefficient of 0.98. Figure 3b,c shows typical time courses of the fluorescent signals of Alexa 488 after α-hemolysin injection, where the fluorescent intensity decay represented passive transport of fluorescent dye molecules through α-hemolysin pore. The average rate constant of the fluorescent decay determined by the fitting with an exponential function (black line in Fig. 3c ) was proportional to the concentration of α-hemolysin in the flow cell (inset in Fig. 3d ), as expected [15] . As a control experiment, we conducted a passive transport assay using Qdot 605 ( φ =10–20 nm), a fluorescent dye larger than the pore size of α-hemolysin that should therefore not be able to pass through the nanopore. As expected, any obvious fluorescent intensity decay was not observed ( Supplementary Fig. 11 ), supporting the validity of the α-hemolysin transport assay. Here, it should be noted that when we injected the excess amount of α-hemolysin (10 μg ml −1 ), most of the microchambers on ALBiC exhibited the α-hemolysin activity (number of active chambers: 11,326 versus total number of sealed chambers: 11,352, yielding 99.8% efficiency). This observation ensured that over 99% of lipid membranes on ALBiC were unilamellar bilayers. Figure 3: Passive transport of fluorescent dye by α-hemolysin. ( a ) Schematic illustration of passive transport of α-hemolysin reconstituted into ALBiCs. The fluorescent dye (Alexa 488) diffused out from the chamber via the hole on the membrane formed by α-hemolysin. ( b ) Fluorescent images of the passive transport activity in the chambers. The images were recorded just after α-hemolysin injection (left panel) and 3,000 s later (middle panel). The right panel, diff., shows the intensity difference between these two images in the form of a colour gradient. ( c ) Continuous recording of the passive transport activity of 1 μg ml −1 α-hemolysin. The average of four representative chambers containing 0 α-hemolysin pores, that of four chambers containing 1 α-hemolysin pore, that of four chambers containing 2 α-hemolysin pores and that of four chambers containing 3 α-hemolysin pores were plotted as grey, blue, red and green, respectively. Over the study period, activity was observed as a continuous decrease in the fluorescence concentration, indicating that α-hemolysin was not inactivated temporarily. Solid lines represent the fittings with the single exponential decay: y = C 1 exp(− k ˙ t )+ C 2 , where k is the rate constant of passive transport. Error bars represent s.d. ( d ) In the histogram, the number of chambers is plotted versus the rate constant of passive transport, k . The four peaks can be attributed to occupancies of 0, 1, 2 or 3 α-hemolysin pores per chamber. They were fitted to a sum of Gaussians. The inset is the average (Ave.) rate constant (const.) against the concentration of α-hemolysin in the flow cell. The grey solid line represents the linear fitting with a correlation coefficient of 0.98. Full size image Next we explored the feasibility of single-molecule detection of α-hemolysin transporting activity. When α-hemolysin was introduced at a lower concentration (that is, 1 μg ml −1 ), the response of each individual chamber was no longer homogeneous ( Fig. 3b ), supporting the stochastic formation of α-hemolysin heptamers in lipid bilayers. Real-time recording of the passive transport by 1 μg ml −1 α-hemolysin revealed a quantization in the rate of fluorescent decay ( Fig. 3c ). The distribution of the rate constants exhibited four distinctive peaks ( Fig. 3d ), suggesting that each peak corresponded to the incorporation of 0, 1, 2 or 3 α-hemolysin pores. The intervals between the peaks were essentially constant, supporting the above conclusion. For further confirmation, we conducted the same assay with diluted α-hemolysin (0.1 μg ml −1 ). The histogram of the transportation rates exhibited only two distinctive peaks ( Supplementary Fig. 12 ). These peaks corresponded to those of 0 and 1 α-hemolysin pore activity obtained at 1 μg ml −1 ; there are no other peaks corresponding to 2 or 3 pores. The proportion of active chambers significantly decreased relative to the proportion of empty chambers. These are typical features of single-molecule digital counting; the concentration of the target molecule only governs the fraction of positive reactors, while the signal from positive reactors containing a single target molecule is constant according to the target concentration. Thus, we concluded that the second peak from the left in Fig. 3d corresponded to the activity of a single α-hemolysin pore. The rate constant of the passive diffusion through a single α-hemolysin pore ( k 1 ) was determined from the peak interval to be 5.5±1.5 × 10 −4 s −1 . The initial transport flux of a single α-hemolysin pore ( v ) was estimated as v = n ˙ k 1 , where n is the number of fluorescent dye molecules encapsulated in each chamber, and n =7 fL × 1 μM × N A =4.2 × 10 3 molecules. The initial transport flux per α-hemolysin pore, as determined under the present conditions, was 2.3 molecules per second, which was much smaller than the detection limit of conventional electrochemical measurements (~10 7 ions per second). Thus, the ALBiC system achieved the highly sensitive detection of passive molecular transport by α-hemolysin. Single-molecule analysis of active membrane transport Next we explored the possibility of single-molecule analysis of the active proton-transporter protein, F 0 F 1 -ATP synthase (F 0 F 1 ). This enzyme mediates energy conversion between the phosphoryl group transfer potential of ATP and proton motive force (PMF) across membranes via mechanical rotation of the inner rotor subcomplex [16] , [17] , [18] , [19] , [20] , [21] , [22] . When the PMF is small or diminishes, F 0 F 1 hydrolyses ATP, actively pumping protons to form PMF. Under physiological conditions where PMF is sufficient, proton flux down PMF forces F 0 F 1 to work in the reverse direction, inducing ATP synthesis. Although extensive single-molecule studies have been conducted for F 0 F 1 , some of the basic features of F 0 F 1 , such as proton conductance and the maximum rate of proton pumping, still remain unclear. In this study, RhP-M was used as a fluorescent pH indicator ( Fig. 4a ) because RhP-M has some technical advantages over other pH-sensitive dyes, including fluorescent enhancement on acidification, a large dynamic range, slow photobleaching and low membrane permeability. Reconstituted liposomes were prepared with a limiting amount of F 0 F 1 to carry only a few molecules (0, 1 or 2 molecules) of F 0 F 1 . When the liposome solution was introduced into the flow chamber, some of the liposomes were fused with the lipid bilayer of ALBiCs, transferring F 0 F 1 molecules to the bilayers ( Fig. 4a ). Then, ATP was injected to initiate proton pumping. In this setup, only F 0 F 1 molecules outwardly orienting the catalytic core domain of F 1 could hydrolyse ATP to pump protons into the chambers ( Fig. 4a ). Inwardly oriented F 0 F 1 molecules did not interfere with the result because F 0 F 1 molecules do not passively transport protons unless a large PMF, typically over 150 mV, is charged on the membrane. 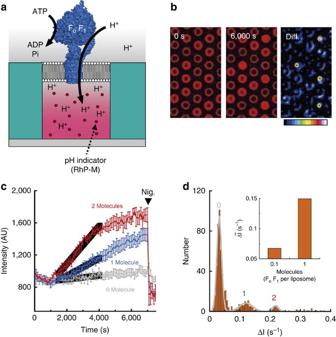Figure 4:Active transport of protons byF0F1-ATP synthase (F0F1). (a) Schematic illustration of F0F1active transport. F0F1pumps the proton from outside to inside the microchamber by hydrolysing ATP. The fluorescent pH indicator (RhP-M) is encapsulated in the microchamber for pH monitoring. (b) Fluorescence images of the proton pumping of F0F1in the chambers. The images were recorded just after the injection of 200 μM ATP (left panel) and 6,000 s later (middle panel). The right panel, diff., shows the intensity difference between the left and middle panels in the form of a colour gradient. (c) Continuous recording of proton pumping. The average of 12 representative chambers containing 0 molecules, that of 12 chambers containing 1 molecule and that of 12 chambers containing 2 molecules of active F0F1were plotted as grey, blue and red, respectively. Over the study period, activity was observed as a continuous increase in fluorescence intensity. Black solid lines represent the linear fittings. Error bars represent s.d. (d) In the histogram, the number of chambers is plotted versus the slope of fluorescence increments from 1,500 to 4,000 s. The three peaks can be attributed to occupancies of 0, 1 or 2 active F0F1molecules per chamber. They were fitted to a sum of Gaussians. The inset is the average slope of fluorescence increments against the average number of active F0F1molecules reconstituted in a single liposome. Figure 4b,c displays typical time courses of fluorescent images obtained after the ATP injection. Similar to the fluorescence signals obtained from the single-molecule α-hemolysin assay, fluorescent signals for F 0 F 1 assays showed heterogeneity. As expected, the differential image in Fig. 4b (left) exhibited discrete signal levels, indicating the stochastic reconstitution of F 0 F 1 molecules. The active chambers reached a plateau at ~1,600, which corresponded to a pH of ~5.4 ( Supplementary Fig. 5 ). The generated transmembrane proton gradient (ΔpH) was ~1.7, which was at a level of equilibrium with the free energy of ATP hydrolysis. At the end of the observation period, an ionophore of H + , nigericin (arrow in Fig. 4c ), was injected into the flow channel. Active chambers always recovered the original fluorescence level. This nigericin-induced fluorescence recovery ensured that the fluorescence increase represented the ATP-driven proton-pumping activity of F 0 F 1 , rather than artefacts, such as spontaneous dissociation of RhP-M from the device wall. For further confirmation, we tested the effects of a specific inhibitor of F 0 F 1 , N , N′ -dicyclohexylcarbodiimide (DCCD) [23] , [24] , which completely blocks the proton-pumping activity of F 0 F 1 . When treated with 10 μM DCCD, F 0 F 1 did not show any detectable activity ( Supplementary Fig. 13 ), supporting the validity of the experiment. Here it should be noted that the aforementioned F 0 F 1 assays were conducted using DOPE and DOPG as lipid components of ALBiC. When we used soy lipid instead of DOPE and DOPG, any fluorescence increments due to proton pumping by F 0 F 1 were not detected, suggesting that the lipid composition can be important for measuring the transport activity of membrane proteins as previously reported [25] . Figure 4: Active transport of protons by F 0 F 1 -ATP synthase ( F 0 F 1 ). ( a ) Schematic illustration of F 0 F 1 active transport. F 0 F 1 pumps the proton from outside to inside the microchamber by hydrolysing ATP. The fluorescent pH indicator (RhP-M) is encapsulated in the microchamber for pH monitoring. ( b ) Fluorescence images of the proton pumping of F 0 F 1 in the chambers. The images were recorded just after the injection of 200 μM ATP (left panel) and 6,000 s later (middle panel). The right panel, diff., shows the intensity difference between the left and middle panels in the form of a colour gradient. ( c ) Continuous recording of proton pumping. The average of 12 representative chambers containing 0 molecules, that of 12 chambers containing 1 molecule and that of 12 chambers containing 2 molecules of active F 0 F 1 were plotted as grey, blue and red, respectively. Over the study period, activity was observed as a continuous increase in fluorescence intensity. Black solid lines represent the linear fittings. Error bars represent s.d. ( d ) In the histogram, the number of chambers is plotted versus the slope of fluorescence increments from 1,500 to 4,000 s. The three peaks can be attributed to occupancies of 0, 1 or 2 active F 0 F 1 molecules per chamber. They were fitted to a sum of Gaussians. The inset is the average slope of fluorescence increments against the average number of active F 0 F 1 molecules reconstituted in a single liposome. Full size image To estimate the proton transport rate of F 0 F 1 at the initial phase where the kinetic effect of PMF was small, the initial rate was measured from the linear portion in the time course (typically from 1,500 to 4,000 s) where fluorescence increased at a constant rate ( Fig. 4c , black lines). The time lag before the linear increment was due to the buffering effect of the solution, masking the transported protons. The averaged proton-pumping rate increased when the amount of F 0 F 1 per liposome increased ( Fig. 4d , inset). The histogram of the proton-pumping rate obtained at the ratio of F 0 F 1 /liposome of 0.1 exhibited three distinct, regularly spaced peaks, indicating that each peak represented chambers with 0, 1 or 2 molecules of active F 0 F 1 . The rate of proton pumping by F 0 F 1 was estimated from the intervals between the peaks to be 27.5 s −1 (see Methods). In the past two decades, various techniques using femtolitre chamber systems have been developed for single-molecule analysis of enzymes [6] , [8] , [9] and have subsequently been applied to digital counting in diagnostic applications [26] , [27] , [28] . The ALBiC system described here broadens the versatility of femtolitre chamber assays to membrane protein analysis. This new platform allows us to form millions of microchambers, each sealed with a lipid bilayer, with high reproducibility and in a high-throughput manner. The formed lipid bilayer was stable and not permeable to fluorescent dyes and ions, demonstrating superiority to conventional lipid bilayer systems such as liposomes or supported lipid bilayers [21] , [29] , [30] , [31] , [32] . The use of an ultra-small reaction chamber dramatically improved detection sensitivity, which allowed the measurement of transport activity of α-hemolysin and F 0 F 1 at the single-molecule level. Thus, the ALBiC system has proven to be a powerful experimental platform for the quantitative analysis of membrane transporters. In this study, we also developed a single-molecule transporter assay for α-hemolysin, in which we detected the transport activity of α-hemolysin as an exponential decay of fluorescent signal. For quantitative analysis, we constructed a simple physicochemical model where we assumed that diffusion of the dye molecules (Alexa 488) through a nanopore of the α-hemolysin molecule was the kinetic bottleneck and obeyed Fick’s law (see Methods). This simple model accurately reproduced the experimental data ( Fig. 3c,d ) and allowed us to estimate the diffusion coefficient of Alexa 488 in the nanopore of α-hemolysin. The estimated diffusion coefficient of Alexa 488 was 5.1 × 10 −11 m 2 s −1 , which was only 8.6 times smaller than the diffusion coefficient of Alexa 488 in free aqueous solution, 4.4 × 10 −10 m 2 s −1 (ref. 33 ). Taking into account that the pore size was comparable to the size of Alexa 488, the reduced diffusion coefficient of Alexa 488 in α-hemolysin pore was reasonable. Indeed, similar or greater reductions in the effective diffusion coefficients of ions have been reported for ion channels [34] , [35] . We also demonstrated the single-molecule analysis of the proton-pumping activity of F 0 F 1 , which had not been achieved before. The proton-pumping rate of single molecule of F 0 F 1 was 27.5 protons per second from the initial linear region of the time course. This is essentially consistent with the previous estimation [36] , reported to be 15–30 protons per second. Because the coupling ratio of protons/turns in bacterial F 0 F 1 is 10 (refs 37 , 38 ), the observed proton-pumping rate corresponds to a rotational rate of 2.8 r.p.s. The resulting ATP hydrolysis rate is 8.4 turnovers per second based on the coupling ratio of ATP per turn=3 (ref. 39 ). The estimated ATP hydrolysis rate was obviously slower than that of detergent-solubilized F 0 F 1 , which has been measured to be ~300 s −1 (ref. 40 ). This is attributable to differences in the conditions under which the assays were conducted; when embedded in the lipid bilayer, F 0 F 1 has to rotate against a much more viscous fluid than in aqueous solution. This would limit the rotational rate, thereby reducing the catalytic rate. Because the reconstitution of F 0 F 1 into the lipid bilayer tightens the rotor–stator interaction [41] , it is also possible that the internal friction between the rotor and stator parts of the F o motor limits the rotational and catalytic rates. The ALBiC system may be applicable as a universal platform to study other transporters, receptors and more complex biosystems that normally function on a lipid bilayer, such as receptor-induced signal transduction and membrane fusion or fission. The ALBiC system should also be applicable for the encapsulation of artificial cell-like systems comprising subcellular systems such as gene transcription and translation, genome replication or some metabolic cascades. The regularly shaped structure and stability of ALBiCs would facilitate the quantitative analysis of such artificial cell systems. In addition, the high-throughput feature of the ALBiC system may also allow for its application in pharmacological screening. On the other hand, the currently developed ALBiC system has several limitations. First, the reaction volume is still too large for slow membrane transporters. In the present work, it took over 1,000 s to detect the proton-pumping activity of single F 0 F 1 molecules. To shorten the detection time, attolitre-scaled ALBiC systems will be required. The shortening of detection time would also enhance detection sensitivity and help to avoid possible artefacts such as photobleaching. Integration with electric systems for charging membrane voltage will also be required because biomembranes generally have electrochemical potential under physiological conditions, driving many transporter proteins and other membrane systems. These points represent remaining technical challenges for further developments of the ALBiC system. Microfabrication We fabricated hydrophobic through-hole structures on a hydrophilic glass substrate using conventional photolithography [27] . A carbon–fluorine hydrophobic polymer (CYTOP, Asahi-glass) was spin coated on a clean cover glass (32 mm × 24 mm) at 4,000 r.p.m. for 30 s and then baked for 1 h at 180 °C. The thickness of the CYTOP layer was 0.5 μm. Photolithography was conducted using a positive photoresist (AZP4903, AZ Electronic Materials, Japan) to pattern mask structures on the CYTOP layer. The resist-patterned substrate was dry etched with O 2 plasma using a reactive-ion etching system (RIE-10NR, Samco, Japan) to expose an array of hydrophilic SiO 2 on the glass surface. The substrate was then cleaned and rinsed with acetone and ethanol to remove the photoresist layer remaining on the substrate. Because the fabrication process was well established, we were able to efficiently fabricate hydrophobic through-hole structures on a hydrophilic glass substrate, achieving a fabrication success rate of 100%. Figure 1 depicts a fabricated device, where the diameter of the CYTOP well is 4 μm. Expression and purification of F 0 F 1 RA1 strain E. coli (unc − /cyo − ) was transformed with the EF 0 F 1 plasmid. After preculture in 5 ml of Lysogeny Broth containing 30 μg ml −1 chloramphenicol for 8–9 h at 37 °C, the cells were inoculated in 1.2 l of Terrific Broth containing 30 μg ml −1 chloramphenicol and then cultured for 16 h at 37 °C. To prepare the inverted membrane vesicles, the cells were collected and washed with buffer containing 100 mM HEPES-KOH (pH 7.5) and 50 mM KCl. The pellet was then resuspended in buffer A (100 mM HEPES-KOH (pH 7.5), 1 mM EDTA, 500 mM sucrose, 1 mM dithiothreitol and 2 × protease inhibitor mixture (Complete, Roche, Switzerland)). Egg-white lysozyme (8–12 mg, Seikagaku, Japan) was added, and the mixture was incubated at room temperature for 20 min. Subsequently, 1–2 mg of DNase I (Roche) and 5 mM MgCl 2 were added, and incubation was carried out at 4 °C for 20 min. The spheroplasts were then spun down, resuspended in buffer B (50 mM HEPES-KOH (pH 7.5), 0.5 mM EDTA, 250 mM sucrose, 0.5 mM dithiothreitol, 5 mM MgCl 2 and 5 mM 4-aminobenzamidine dihydrochloride (PAB)) and sonicated on ice. They were then centrifuged at 9,000 r.p.m. for 10 min at 4 °C to remove the cell debris. The supernatant containing the inverted membrane was transferred to a new tube and centrifuged at 75,000 r.p.m. for 20 min at 4 °C. The supernatant was discarded, and the pellet was resuspended in buffer B at 250 mg ml −1 . To purify EF 0 F 1 , the membrane suspension (250 mg ml −1 , wet weight of inverted membrane/volume of buffer) in 0.8% (w/v) n-octyl β- D -glucopyranoside (Sigma, USA) was centrifuged at 75,000 r.p.m. for 20 min at 4 °C. The pellet was transferred to a new tube on ice. Buffer C (20 mM HEPES-KOH (pH 7.5), 500 mM NaCl, 5 mM MgCl 2 , 200 μM ADP, 50 mM imidazole, 20% (v/v) glycerol, 1 × protease inhibitor mixture and 5 mM PAB) and 2% (w/v) octaethylene glycol mono-n-dodecyl ether (C12E8, Wako, Japan) were added to the pellet, and the mixture was incubated for 15 min on ice. It was then centrifuged, and the supernatant was collected. The collected supernatant was injected into a HisTrap HP column (GE Healthcare, UK) pre-equilibrated with 5 ml of buffer D (20 mM HEPES-KOH (pH 7.5), 500 mM NaCl, 5 mM MgCl 2 , 200 μM ADP, 50 mM imidazole, 20% glycerol (v/v), 1 × protease inhibitor mixture, 5 mM PAB, 0.3% (w/v) C12E8 and 0.1% (w/v) E. coli total lipid (Avanti, USA)). The column was washed twice with 5 ml of buffer D. His-tagged EF 0 F 1 was eluted with 3 ml of buffer E (20 mM HEPES-KOH (pH 7.5), 500 mM NaCl, 5 mM MgCl 2 , 200 μM ADP, 500 mM imidazole, 20% glycerol (v/v), 1 × protease inhibitor mixture, 5 mM PAB, 0.3% (w/v) C12E8 and 0.1% (w/v) E. coli total lipid). Six drops of the eluate were collected in each 1.5-ml tube containing 1 mM dithiothreitol. The purified EF 0 F 1 fractions were run on 15% SDS–polyacrylamide gel electrophoresis to select the purest fractions that contained all the subunits and the least contaminants. The chosen fractions were pooled and passed through a NAP-5 column (GE Healthcare) that had been pre-equilibrated with buffer F (20 mM HEPES-NaOH (pH 7.5), 100 mM NaCl, 2 mM MgCl 2 , 0.1 × protease inhibitor mixture, 5 mM PAB, 0.3% (w/v) C12E8 and 0.1% (w/v) E. coli total lipid). EF 0 F 1 was eluted with 1 ml of buffer F. The eluate was concentrated and further purified in an Amicon Ultra-4 100,000 centrifugal filter device (Millipore, USA). The protein concentration of the sample was determined by the BCA assay (Thermo Fisher Scientific, USA) using bovine serum albumin (Sigma) as the standard. Purified EF 0 F 1 was immediately used for reconstitution into the liposome. Imaging Fluorescent time-lapse recordings were taken under a confocal microscope system with a × 60 objective lens and photomultiplier tubes (A1R, Nikon, Japan). Two types of lasers were used for the excitation of Alexa 488 ( λ ex =488 nm), RhP-M ( λ ex =561 nm), Fluo-3 ( λ ex =488 nm) and Qdot 605 ( λ ex =488 nm). The fluorescence intensity was recorded through a × 60 objective lens with photomultiplier tubes (Nikon). Analysis was performed using NIS Elements software (Nikon). Bright-field images of lipid membrane formation were taken under an optical microscope with a × 100 objective lens (IX 71, Olympus, Japan). Photobleaching experiment In the Alexa 488 (Life Technologies, USA) and RhP-M experiments, the flow cell and microchambers were filled with buffer G (100 μM HEPES (pH 7.1), 20 mM NaCl, 2 mM MgCl 2 ) and buffer G containing 1 μM Alexa 488 or buffer G and buffer G containing 10 μM RhP-M, respectively. Using the laser-scanning system of the confocal microscope, one of the chambers was photobleached for a few seconds. The fluorescent images were recorded at 100-s intervals. Ion-leakage experiment The flow cell and microchambers were initially filled with buffer H at pH 5.0 (1 mM MES (pH 5.0), 20 mM NaCl, 2 mM MgCl 2 ). A pH probe, RhP-M, was also introduced into the inside of the microchambers at 10 μM. Then, buffer H (1 mM HEPES (pH 7.1), 20 mM NaCl, 2 mM MgCl 2 ) was introduced into the flow cell. The fluorescent images of RhP-M were recorded at 100-s intervals for 2 h. For evaluation of possible Ca 2+ leakage, the flow cell and microchambers were initially filled with buffer I (1 mM HEPES (pH 8), 100 μM CaCl 2 , 20 mM NaCl, 2 mM MgCl 2 ). The microchambers were also loaded with a Ca 2+ indicator Fluo-3 at 20 μM. Then, buffer I in the flow cell was exchanged with buffer J (1 mM HEPES (pH 8), 100 nM CaCl 2 , 20 mM NaCl, 2 mM MgCl 2 ). After buffer exchange, the fluorescent images of Fluo-3 were recorded at 300-s intervals for 2 h. Biological assays in the chambers To examine passive transport by α-hemolysin (Sigma Aldrich, USA), the flow cell and microchambers were filled with buffer G and buffer G containing 1 μM Alexa 488 or 100 nM Qdot 605 (Life Technologies), respectively. After lipid membrane formation, a certain amount of α-hemolysin was injected into the flow cell. To examine proton pumping by F 0 F 1 , the flow cell and microchambers were filled with buffer G and buffer G containing 10 μM RhP-M, respectively. To reconstitute F 0 F 1 into the lipid bilayers, we injected a solution containing F 0 F 1 -reconstituted liposomes and 5% polyethylene glycolinto the flow cell and incubated the samples for 30 min. After the reconstitution of F 0 F 1 into the lipid bilayers, buffer G containing 240 μM ATP was injected into the flow cell. Fluorescence images were recorded at 20- or 100-s intervals for α-hemolysin and F 0 F 1 , respectively. Analysis of passive transport of Alexa 488 by α-hemolysin To reproduce the experimental results depicted in Fig. 3c , we constructed a physical model of α-hemolysin based on Fick’s law. The nanochambers were filled with buffer G containing 1 μM Alexa 488. The passive transport of Alexa 488 can be written as follows: where N , V , C in ( t ), J Alexa ( t ) and d are the number of α-hemolysin molecules reconstituted in the chamber, volume of the chamber (7 fL), concentration of Alexa 488 in chamber, passive transport rate and diameter of the α-hemolysin pore ( d =~1 nm), respectively. The size of the chamber was relatively small compared with the diffusion rate of Alexa 488, and therefore the rate-limiting step of passive transport was the translocation of Alexa 488 through the α-hemolysin pore, which can be written using Fick’s law: where D and L are the diffusion coefficient of Alexa 488 and the length of the α-hemolysin pore ( L =~10 nm), respectively. Then, from equations (1) and (2), the passive transport can be written as Initial condition: C in ( t )= C 0 at t =0. The differential equation was solved, and C in ( t ) was expressed by In the present study, the fluorescent intensity of Alexa 488 was proportional to its concentration ( Supplementary Fig. 3 ), and therefore the fluorescent intensity of Alexa 488 encapsulated in the chamber, that is, F ( t ), was expressed by The observed time courses of passive transport were well fitted to equation (5) ( Fig. 3c ), allowing us to estimate the diffusion coefficient of Alexa 488 in the nanopore of α-hemolysin as 5.1 × 10 −11 m 2 s −1 , which was the only fitting parameter in equation (5). Analysis of proton pumping by F 0 F 1 To reproduce the experimental results depicted in Fig. 4c , we constructed a physicochemical model of proton pumping by F 0 F 1 in ALBiCs ( Supplementary Fig. 14A ). The nanochambers were filled with buffer G containing 10 μM pH indicator. The buffer (HEPES) and RhP-M are sensitive to pH; therefore, their equilibrium can be written as follows: where [B − ], [In − ], [BH] and [InH] are the concentrations of buffer, RhP-M and the generic acids of buffer and RhP-M, respectively. Because the volume of the nanochamber is so small, the chemical species are supposed to be in equilibrium. Therefore, the acid dissociation constants, and , are written as a quotient of the concentrations of chemical species as follows: where and are determined as 10 −7.4 and 10 −6 M, respectively ( Supplementary Fig. 5 ). Then, the balance of protons in a chamber is given by: where J ( t ), N A and V are the proton-pump rate of F 0 F 1 , Avogadro constant and volume of the nanochamber, respectively. The initial conditions of and V were 10 −7.1 M and 7 fL, respectively. Then, assuming J ( t ) was constant, simultaneous equations (5)–(7), ,  were solved. From the titration curve shown in Supplementary Fig. 5 , the fluorescent intensity of RhP-M is expressed as follows: As shown in Supplementary Fig. 14 , the time courses of proton pumping by F 0 F 1 ( Fig. 4c ) were well fitted with the function equation (8), only requiring the fitting parameter J ( t ). J ( t ) values determined for a single molecule or two molecules of F 0 F 1 were 30 and 50 s −1 , respectively, from which the proton pump rate of a single molecule of F 0 F 1 was determined to be 27.5 s −1 . How to cite this article: Watanabe, R. et al. Arrayed lipid bilayer chambers allow single-molecule analysis of membrane transporter activity. Nat. Commun. 5:4519 doi: 10.1038/ncomms5519 (2014).